Strong plasmonic enhancement of photovoltage in graphene From the wide spectrum of potential applications of graphene, ranging from transistors and chemical sensors to nanoelectromechanical devices and composites, the field of photonics and optoelectronics is believed to be one of the most promising. Indeed, graphene's suitability for high-speed photodetection was demonstrated in an optical communication link operating at 10 Gbit s −1 . However, the low responsivity of graphene-based photodetectors compared with traditional III–V-based ones is a potential drawback. Here we show that, by combining graphene with plasmonic nanostructures, the efficiency of graphene-based photodetectors can be increased by up to 20 times, because of efficient field concentration in the area of a p–n junction. Additionally, wavelength and polarization selectivity can be achieved by employing nanostructures of different geometries. The unique optical and electronic properties of graphene [1] , [2] make it ideal for a number of photonic applications [3] , [4] , [5] , [6] , [7] . In particular, graphene-based photodetectors have excellent characteristics in terms of quantum efficiency and reaction time, because of the very large room-temperature mobility and high Fermi velocity of charge carriers in this material [8] , [9] , [10] . Although the exact mechanism for light to current conversion is still debated [11] , [12] , a p–n junction is usually required to separate the photo-generated electron–hole pairs. Such p–n junctions are often created close to the contacts, because of the difference in the work functions of metal and graphene [13] , [14] . Whatever the photocurrent generation mechanism, all such devices suffer from several problems, such as low light absorption of graphene (2.3% of normal incident light [15] , [16] ); difficulty of extracting photoelectrons (only a small area of the p–n junction contributes to current generation); and the absence of a photocurrent for the condition of uniform flood illumination on both contacts of the device. Unless the contacts are made of different materials, the voltage/current produced at both contacts will be of opposite polarity for symmetry reasons, resulting in zero net signal [8] , [10] , [11] . One possible way of overcoming these restrictions is to utilize plasmonic nanostructures placed near the contacts. Incident light, absorbed by such nanostructures, can be efficiently converted into plasmonic oscillations, which leads to a dramatic enhancement of the local electric field. One might consider this process as generation of evanescent photons that exist only in the near-field region [17] , [18] , [19] , [20] . Such a field enhancement, exactly in the area of the p–n junction formed in graphene, can result in a significant performance improvement of graphene-based photodetectors. The role of the suggested plasmonic nanostructures is therefore to guide the incident electromagnetic energy directly to the region of the p–n junction. Here we demonstrate that the efficiency of nanostructured devices of this kind can be 20 times larger than that of traditional devices [8] , [9] , [10] . Sample design We used graphene prepared by micromechanical exfoliation of graphite [21] , [22] . The single-layer nature of our flakes was confirmed by a combination of optical contrast [23] , [24] , [25] , Raman spectroscopy [26] and quantum Hall effect [27] , [28] measurements. Ti/Au (3 nm Ti, 80 nm Au) contacts were formed by e-beam lithography, e-beam evaporation and lift-off. 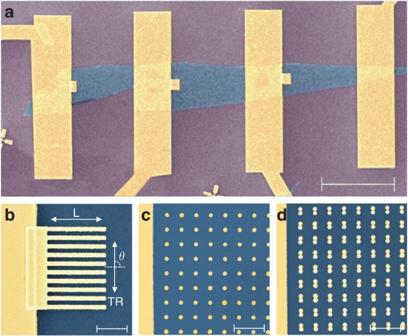Figure 1: Scanning electron microscopy micrographs of the graphene devices with plasmonic nanostructures. (a) An overall image of one of our devices (in false colours). Blue, graphene; purple, SiO2(300 nm); yellow, Ti/Au electrodes. Scale bar, 20 μm. (b–d) Blow up of contacts with various tested plasmonic nanostructures (in false colours). L and TR incident light polarizations are indicated. Scale bar, 1 μm. Figure 1a shows the layout of the resulting devices. Various nanostructures were fabricated close to the macroscopic contacts of such two-terminal devices (examples are shown in Fig. 1b–d ). The layout and composition of the structures are chosen to produce strong light absorption in the visible range, and are similar to what we previously designed to achieve a plasmonic blackbody, resulting in almost complete absorption of incident visible light [29] . We employed several different designs, but here we will mainly concentrate on one particular structure (grating with 110 nm finger width, 300 nm pitch, Fig. 1b ), which showed the best performance. Figure 1: Scanning electron microscopy micrographs of the graphene devices with plasmonic nanostructures. ( a ) An overall image of one of our devices (in false colours). Blue, graphene; purple, SiO 2 (300 nm); yellow, Ti/Au electrodes. Scale bar, 20 μm. ( b – d ) Blow up of contacts with various tested plasmonic nanostructures (in false colours). L and TR incident light polarizations are indicated. Scale bar, 1 μm. Full size image Electrical characterization The local photovoltage and photocurrent response of our devices is measured by coupling several lasers to a microscope, as described in Methods, and by scanning the position of the illumination spot. This allows us to measure the photovoltage dependence on intensity, wavelength and polarization of the incoming light, as well as the gate voltage. The laser power on the samples is kept at ∼ 30 μW. At this power, the photovoltage signal is larger than any thermopower-related signal (verified by changing the incident power). This laser intensity is also low enough not to result in any observable overheating of the samples (which ensures that we work in the linear regime). Our devices have reasonable field effect mobility ∼ 5,000 cm 2 V −1 s −1 at room temperature ( Fig. 2a ). They show unintentional p-doping of up to 5×10 12 cm −2 (confirmed both by electronic transport [30] and Raman measurements [31] , [32] , Fig. 2c,d ), probably because of water adsorption [30] . 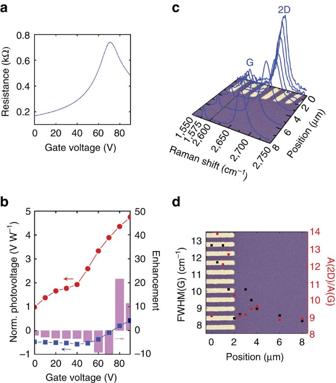Figure 2: Resistance and photovoltaic characteristics. (a) Resistance as function of the gate voltage. (b) Normalized photovoltage for illumination close to the FC (blue), close to the SC (red) and enhancement (purple) as function of the gate voltage. Illumination wavelength 514 nm. (c) Raman spectra recorded on graphene at different distances from the SC. (d) FWHM(G) and A(2D)/A(G) as a function of position. The contacts provide local weak p-type doping [14] , again confirmed by the Raman data, Figure 2c,d . The photovoltage generated on the non-structured, flat part of the contact (FC), is positive for electron doping, and negative for hole doping, as a consequence of the formation of p–n or p − –p + junctions, see Figure 2b . Figure 2: Resistance and photovoltaic characteristics. ( a ) Resistance as function of the gate voltage. ( b ) Normalized photovoltage for illumination close to the FC (blue), close to the SC (red) and enhancement (purple) as function of the gate voltage. Illumination wavelength 514 nm. ( c ) Raman spectra recorded on graphene at different distances from the SC. ( d ) FWHM(G) and A(2D)/A(G) as a function of position. Full size image Photovoltage measurements The photovoltage generated on the structured part of the contact (SC) is significantly higher than that on the FC. The enhancement is more than one order of magnitude for the case of the p–n junction ( Fig. 2b ). However, the photovoltage generated on the SC has remarkably different behaviour than that on the FC. It is positive for all the gate voltages measured, monotonically decreasing for higher hole doping, Figure 2b . We do not have a complete understanding of this phenomenon, but we speculate that the most probable reason is the complex distribution of the optical electric field around the SC, which allows us to probe different parts of the p–n or p − –p + junctions in comparison with the FC. The doping profile is confirmed by a Raman line scan across the contacts, carried out at zero gate voltage, Figure 2c . Figure 2d plots the ratios of the areas of 2D and G peaks, A(2D)/A(G), and the full width at half maximum of the G peak, FWHM(G). Far away from the contacts, the Raman parameters correspond to ∼ 5×10 12 cm −2 p-doping [31] , [32] ( Fig. 2d ), consistent with the transport gate-voltage measurements ( Fig. 2a ). A(2D)/A(G) significantly increases when moving close to the contacts, accompanied by a FWHM(G) increase. This implies the sample becomes less p-doped, with the area around contacts being only lightly p-doped, up to about few 10 11 cm −2 (refs 31 , 32 ). In the vicinity of the SC, it can be seen in Figure 2d that both FWHM(G) and A(2D)/A(G) exhibit a non-monotonous behaviour, resulting in local maxima. This can be explained by the interplay between the inhomogeneous doping and strong amplification of the Raman signal around the metallic nanostructures [18] . Photovoltage mapping and polarization dependence To demonstrate the plasmonic nature of the enhancement, we mapped the photovoltaic response for different polarizations and excitation wavelengths for normal light incidence ( Fig. 3 ). This allowed us to directly compare the signal produced when shining light on the FC and SC. Wavelengths covering the visible to near-infrared range (457, 488, 514, 633 and 785 nm, corresponding to Fig. 3a–e , respectively) were used. 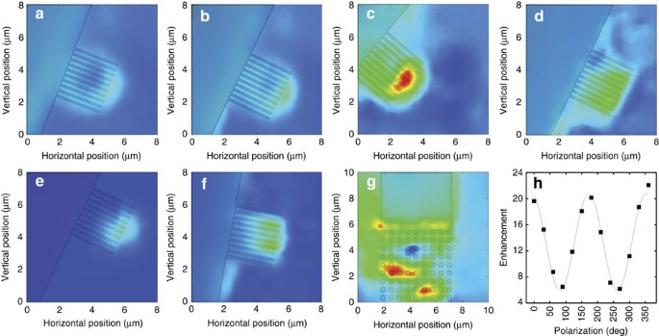Figure 3: Photovoltage maps of one of the nanostructured contacts. The signal (normalized to laser power) measured on a contact with finger structure (finger width 110 nm, pitch 300 nm, except forg) as a function of the position of the illumination spot (spot size∼1.5 μm for various excitation wavelengths. Gate voltage 90 V. Colour scale (except forg), from 0 μV (blue) to 20 μV (red). Overlaid is a schematic position of the contact. (a) 457 nm, TR polarization. (b) 488 nm, TR polarization. (c) 514 nm, TR polarization. (d) 633 nm, TR polarization. (e) 785 nm, TR polarization. (f) 514 nm, L polarization. (g) Example of photovoltage measured on a sample with an array of nanodots; 633 nm, TR polarization. Colour scale, from −4 μV (blue) to 12 μV (red). (h) Polarization-dependent enhancement atλ=514 nm, with 0° being TR polarization. Black squares, measured data; red line, cos2θfit. Figure 3 shows that the SC provides some level of enhancement for all the wavelengths used (the photovoltage on the SC is always larger than that on the FC). The generated photovoltage is usually maximum when the laser beam is positioned at the tips of the nanostructures. This is because, in this area, both large electron band bending (because of doping from the contacts [13] , [14] ) and strong enhancement of the optical field [17] , [18] , [19] , [20] are achieved. In between the metal stripes, although the optical field enhancement is still produced, the band bending is significantly smaller because of screening by the metal contacts. Figure 3: Photovoltage maps of one of the nanostructured contacts. The signal (normalized to laser power) measured on a contact with finger structure (finger width 110 nm, pitch 300 nm, except for g ) as a function of the position of the illumination spot (spot size ∼ 1.5 μm for various excitation wavelengths. Gate voltage 90 V. Colour scale (except for g ), from 0 μV (blue) to 20 μV (red). Overlaid is a schematic position of the contact. ( a ) 457 nm, TR polarization. ( b ) 488 nm, TR polarization. ( c ) 514 nm, TR polarization. ( d ) 633 nm, TR polarization. ( e ) 785 nm, TR polarization. ( f ) 514 nm, L polarization. ( g ) Example of photovoltage measured on a sample with an array of nanodots; 633 nm, TR polarization. Colour scale, from −4 μV (blue) to 12 μV (red). ( h ) Polarization-dependent enhancement at λ =514 nm, with 0° being TR polarization. Black squares, measured data; red line, cos 2 θ fit. Full size image We observed enhancement of the photovoltage for all wavelengths that we measured, with maximum amplification of more than 20 at the plasmonic resonance of our structures. Indeed, the strong spectral dependence of the photovoltaic enhancement suggests the importance of the plasmonic resonances in our nanostructures. The maximum enhancement for 110 nm wide stripes ( Figs. 3 and 4 ) is observed at 514 nm ( Fig. 4a , which is useful for solar cell applications, for instance). Depending on the SC dimensions, the resonance can be tailored to match any part of the spectrum, which might be important for applications in telecommunication. Indeed, for wider structures, the resonance shifts towards larger wavelengths (for example, the 130 nm wide stripes have maximum enhancement close to 633 nm, Fig. 4b ). Such wavelength dependence rules out the possibility that this enhancement is simply because of the geometric enlargement of the junction area for the nanostructured contacts. We note that light interference in SiO 2 can provide some dependence of the photovoltage on the wavelength of the excited light, and can be used to enhance the signal even further [33] . However, in our experiments, the enhancement coefficient ( Fig. 4 ) does not depend on the optical properties of SiO 2 and allows us to concentrate on the performance of such plasmonic nanostructures. 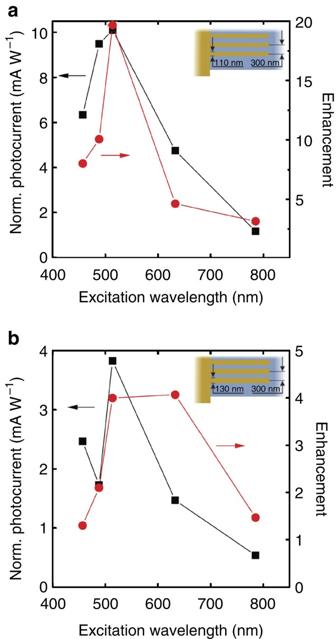Figure 4: Normalized photocurrent and maximum enhancement coefficient. Both characteristics measured as a function of excitation wavelength for two of our finger structures of 300 nm pitch and (a) finger width 110 nm and (b) 130 nm. Insets, schematic representations of such structures. Figure 4: Normalized photocurrent and maximum enhancement coefficient. Both characteristics measured as a function of excitation wavelength for two of our finger structures of 300 nm pitch and ( a ) finger width 110 nm and ( b ) 130 nm. Insets, schematic representations of such structures. Full size image The SC photovoltage polarization dependence can be fitted with a cos 2 θ function, Figure 3h , where θ is the angle between the polarization and the long sides of the nanostructured 'fingers' ( Fig. 1 ). The transverse (TR) polarization gives much stronger enhancement than the longitudinal (L) polarization, as the former couples resonantly to the plasmonic modes across the nanostructured fingers, matching the plasmon wavelength [34] . The FC photovoltage polarization dependence is much weaker (the difference between TR and L does not exceed 30%). We stress that, although the far-field polarization properties of the metal stripes also show cos 2 θ dependence, they cannot be responsible for the enhancement of photovoltage compared with the FC. Hence the observed large anisotropy in enhancement ratio comes from the near-fields generated by plasmonic nanoresonators. We modelled the enhancement of the electric field with the help of finite element analysis using the High Frequency Structure Simulator (HFSS11) [35] . The actual device geometry was utilized in the model, and the optical constants of gold, graphene and the substrate were taken from ref. 29 . 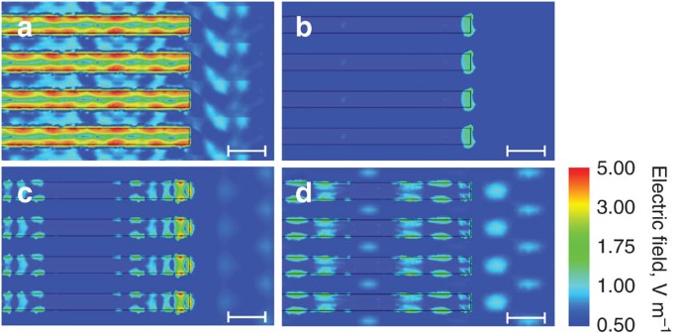Figure 5: Numerical finite element simulations of local electric field. (a) 514 nm, TR polarization. (b) 514 nm, L polarization. (c) 633 nm, TR polarization. (d) 633 nm, L polarization. Scale bar, 300 nm. Figure 5 shows the amplitude of the in-plane electric field around the nanostructures for incident light wavelengths of 514 nm ( Fig. 5a,b ) and 633 nm ( Fig. 5b,c ) and TR and L polarizations. The results correlate well with our experimental data, see Figures 3 and 4 . Thus, the TR polarization for 514 nm excitation ( Fig. 5a ) gives very strong field enhancement on 110 nm wide structures: a factor 5 in terms of field, which is a factor 25 in terms of power amplification—very similar to what we observe in our experiment, Figure 4 . The enhancement is much weaker for 633 nm excitation, again in excellent agreement with our experiments. We note, however, that one cannot draw a direct quantitative comparison between the calculated field enhancement and the measured photovoltaic signals. Indeed, the generated photovoltage depends on two factors: the amplitude of the local optical field and the strength and direction of the electronic band bending (built-in electric field because of the p–n junctions). The field amplification is strongly inhomogeneous, increasing strongly near the contact edges, Figure 5a . This, together with the fact that the p–n junction profile might also be non-trivial, complicates the problem. However, the qualitative correspondence between the experimental results and the theoretical predictions proves the viability of the concept of using field amplification by plasmonic nanostructures for light harvesting in graphene-based photonic devices. Figure 5: Numerical finite element simulations of local electric field. ( a ) 514 nm, TR polarization. ( b ) 514 nm, L polarization. ( c ) 633 nm, TR polarization. ( d ) 633 nm, L polarization. Scale bar, 300 nm. Full size image As an additional benefit, nanostructures with geometries resonant at desired wavelengths can be utilized in graphene-based photodetectors for selective amplification, potentially allowing light filtering and detection, as well as polarization determination in a single device at high operating frequencies. The frequency performance can be even improved in comparison with traditional devices, as the plasmonic structures add only negligible contribution to the capacitance (fractions of femto-Farads), but can significantly reduce the contact resistance. We believe that further optimization of such plasmonic nanostructures (for example, making use of coupled or cascaded plasmon resonances [35] , [36] ) might lead to even greater photovoltage enhancement. Device fabrication Graphene was exfoliated from graphite by mechanical cleavage onto Si covered with 300 nm SiO 2 . Subsequently, contacts including nanostructures were fabricated using e-beam lithography, Ti(3 nm)/Au(80 nm) evaporation and lift-off. Fabricated samples were bonded in a chip carrier for characterization. Photovoltage mapping A 2182A Nanovoltmeter (Keithley) was used to record the photovoltage at the device terminals with an additional 2400 Sourcemeter (Keithley), allowing control of the gate voltage. Laser light (457, 488, 514, 633 and 785 nm) generated from multiwavelength Ar+, He–Ne and solid-state infrared lasers was coupled to the sample by using a DM LM microscope (Leica) and a ×100 ultra-long working distance objective, resulting in a ∼ 1.5-μm spot size. A Physik Instrumente piezoelectric stage was used to translate the sample with respect to the laser spot in the x/y directions with 200-nm steps, resulting in position-dependent recording of the generated photovoltage. Measurements were done at room temperature in ambient atmosphere. Raman spectroscopy Raman spectra were collected by coupling the light scattered from the sample to an inVia Raman spectrometer (Renishaw). Spectra are recorded by using a DM LM microscope (Leica) using a ×100 ultra-long working distance objective. The laser power is kept below 1.5 mW to exclude possible heating effects. How to cite this article: Echtermeyer, T. J. et al . Strong plasmonic enhancement of photovoltage in graphene. Nat. Commun. 2:458 doi: 10.1038/ncomms1464 (2011).